Large-scale self-assembled zirconium phosphate smectic layers via a simple spray-coating process The large-scale assembly of asymmetric colloidal particles is used in creating high-performance fibres. A similar concept is extended to the manufacturing of thin films of self-assembled two-dimensional crystal-type materials with enhanced and tunable properties. Here we present a spray-coating method to manufacture thin, flexible and transparent epoxy films containing zirconium phosphate nanoplatelets self-assembled into a lamellar arrangement aligned parallel to the substrate. The self-assembled mesophase of zirconium phosphate nanoplatelets is stabilized by epoxy pre-polymer and exhibits rheology favourable towards large-scale manufacturing. The thermally cured film forms a mechanically robust coating and shows excellent gas barrier properties at both low- and high humidity levels as a result of the highly aligned and overlapping arrangement of nanoplatelets. This work shows that the large-scale ordering of high aspect ratio nanoplatelets is easier to achieve than previously thought and may have implications in the technological applications for similar materials. Large-scale assembly methods are used to create highly aligned fibres of Kevlar, Twaron and carbon nanotubes [1] , [2] , [3] , which show an exceptional combination of light weight, high mechanical strength and additional functional properties such as impact toughness, chemical resistance, electrical conductivity and so on. Such a high degree of order is achieved through the lyotropic character of the constituent structural elements, which can be polymeric mesogens or individual nanotubes. These structural elements can be manipulated to form liquid crystalline phases in solutions, from which continuous fibres may be drawn or spun out. A key feature of this process is that the resulting fibres inherit the orientation and arrangement from the liquid crystalline phase in the parent solution. In recent years, research on two-dimensional (2D) crystals has shown that graphene oxide nanosheets can also be spun into highly aligned fibres using a similar process [4] . Nevertheless, this assembly method has not been shown to be successful in manufacturing materials with form factors other than continuous fibres. The phenomenon of large aspect ratios nanomaterials (including nanorods and nanoplatelets) organizing into mesophases is explained by Onsager’s theory [5] . Onsager accurately described the formation of nematic phases of hard rigid rods at concentrations above the critical volume fraction owing to a small net gain in entropy. As aspect ratios increases, critical volume fraction for the isotropic to nematic transition decreases. The lyotropic behaviour of nanomaterials can be exploited to create large-scale assemblies in the form of coatings that consist of mesoscale structures possessing long-range positional and orientational order. The formation of such structures significantly enhances the performance of the coatings. The self-assembled coatings of α-ZrP (α-zirconium phosphate, Zr(HPO 4 ) 2 ·H 2 O) nanoplatelets/polymer layers are created using a highly efficient process. Liquid crystalline phases of nanoplatelets are typically achieved via the electrostatic repulsion of the charges on the surface of nanoplatelets in aqueous solutions [6] , [7] or sterically stabilized nanoplatelets in organic solutions [8] , [9] . Here we show that sterically stabilized nanoplatelets suspended in organic solution mixed with an appropriate pre-polymer or polymer can preserve the mesomorphic structure of the nanoplatelets even after the solvent is removed. This property allows the formation of a self-assembled smectic layer of nanoplatelets in epoxy via a simple, spray-coating process. We further demonstrate that gas permeability can be easily varied by adjusting nanoplatelet concentration in the nanocomposite film. This effect is correlated to a decrease in inter-layer d -spacing of the nanoplatelets as concentration increases, leading to a higher barrier against gas permeation. Spray-coatable oligomer-tethered nanoplatelets A solution containing a mixture of oligomer-grafted nanoplatelet and polymer is deposited as a continuous film on a substrate using spray-coating ( Fig. 1a,b ). Subsequent drying and removal of solvent induces self-assembly of the smectic phase in the film ( Fig. 1c ). The mesomorphic structure is then stabilized by curing the matrix to form a robust coat of cured epoxy ( Fig. 1d ). This fast, simple process of delivering nanoplatelets to a substrate allows the final film to retain the liquid crystalline order of the nanoplatelets. The usefulness of the mesomorphic nanoplatelets in coatings is demonstrated by measuring the oxygen transmission rates (OTRs) of polyimide (PI) films coated with the smectic α-ZrP nanoplatelet/epoxy nanocomposite. The oxygen permeability of the coated films is significantly reduced compared with the film coated only with epoxy. The effectiveness of the barrier films is a result of small gas molecules being forced to traverse a tortuous path created by impenetrable nanoplatelets ( Fig. 1e ) [10] . 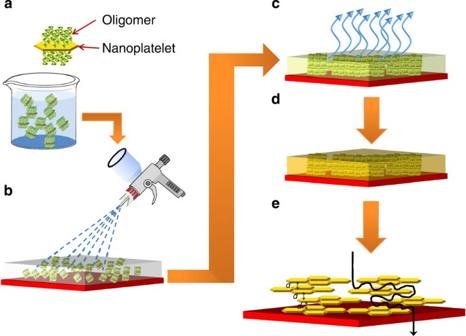Figure 1: Spray-coating of smectic α-ZrP/epoxy films. (a) Oligomer-grafted nanoplatelets are dispersed in a solution with epoxy pre-polymer and curing agent. (b) Solution is sprayed onto a PI substrate. (c) Coated substrate is dried and nanoplatelets self-assemble into smectic phases during solvent evaporation. (d) Nanocomposite is cured to form a robust coat. (e) Gas molecule forced to traverse tortuous path to arrive at other side of barrier film (oligomer and epoxy omitted from schematic for clarity). The inter-layer distancedis constant between each layer. The black line traces a probable diffusion path of a gas molecule. Figure 1: Spray-coating of smectic α-ZrP/epoxy films. ( a ) Oligomer-grafted nanoplatelets are dispersed in a solution with epoxy pre-polymer and curing agent. ( b ) Solution is sprayed onto a PI substrate. ( c ) Coated substrate is dried and nanoplatelets self-assemble into smectic phases during solvent evaporation. ( d ) Nanocomposite is cured to form a robust coat. ( e ) Gas molecule forced to traverse tortuous path to arrive at other side of barrier film (oligomer and epoxy omitted from schematic for clarity). The inter-layer distance d is constant between each layer. The black line traces a probable diffusion path of a gas molecule. Full size image The general concept of using nanoplatelets sterically stabilized by oligomers in combination with a pre-polymer or polymer to fix the mesomorphic structure in the solid state is applicable to 2D crystals. The spray-coating technique allows for fast, efficient application of functional coatings onto a substrate under ambient conditions that potentially offers a scalable approach to create multilayer functional coatings reminiscent of hierarchical structures commonly observed in biology [11] , [12] . α-ZrP has a layered structure and has been studied for many uses [13] , [14] , [15] , [16] , [17] . Relatively strong P-OH Brønsted acid groups in α-ZrP monolayers allow for functionalization with proton donors such as amines, even in solutions of low basic strength [18] , [19] . The intercalation of such ionic species into the inter-layers weakens the inter-layer binding and promotes exfoliation of the layered structures into individual 2D crystals. Liquid exfoliation using similar intercalation methods have been demonstrated in a broad family of layered functional materials such as transition metal oxides [20] and dichalcogenides [21] , layered double hydroxides [22] , h-BN [23] and even graphene [24] , [25] . Thus, it is suggested that liquid exfoliation via surface functionalization using oligomeric compounds is a general method, and the phenomenon observed here should be applicable to these other layered materials with the proper selection of compatible functionalizing species and solvent. Hexagonal nanoplatelets with average size of 100±51 nm ( Fig. 2a ) were synthesized via a hydrothermal method according to Sun et al. [18] Monoamine polyoxyalkyleneamines are effective in exfoliating α-ZrP nanoplatelets in organic solvents such as acetone [19] . A polyoxyalkyleneamine with weight-average molecular weight of about 1,000 (Jeffamine M1000, Huntsman Chemical) was selected and is comparable to oligomers that were used in previous reports [8] , [9] . Atomic force microscopy (AFM) reveals that the exfoliated α-ZrP nanoplatelets (see Methods) are coated with a soft layer ( Fig. 2b,c ). This soft layer is as thick as 10 nm when swollen by butyronitrile, suggesting that a significant amount of free oligomer is adsorbed onto the nanoplatelet. The height of the nanoplatelet lies in the range of 0.5–0.7 nm, in close agreement with the expected value of 0.68 nm from crystallography studies [26] . Spray-coated smectic α-ZrP/epoxy films were prepared on PI (thickness 25 μm Apical, Kaneka). The aspect ratio, α is defined as α = D/t =100/0.68=147, where D is the diameter and t is the thickness [10] , [27] , [28] , [29] . The spray-coated PI films remained highly transparent and flexible after being fully cured ( Fig. 2d,e ). The reported volume fractions are based on inorganic α-ZrP mass exclusively, which was obtained by thermogravimetric analysis (see Methods). 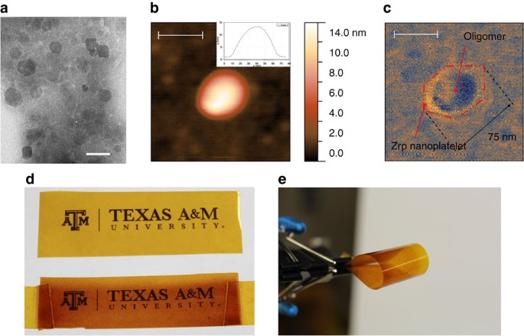Figure 2: α-ZrP nanoplatelets and spray-coated films. (a) Transmission electron microscopy (TEM) of α-ZrP nanoplatelets with average size of 100±51 nm, measured from over 200 particles. Scale bar, 100 nm. (b) Atomic force microscopy (AFM) height image shows a nanoparticle with grafted brush layer swollen with butyronitrile exhibiting a hemispherical shape (10 nm thick; inset, height profile of nanoparticle). (c) Phase image of the same nanoparticle reveals a stiffer phase in the shape of a hexagon at the base (75 nm wide). Scale bar inb,crepresents 50 nm. (d) Photographs of PI film (top, thickness 25 μm) and PI film spray-coated with smectic α-ZrP/epoxy (bottom, coating thickness 8 μm), demonstrating a uniform, transparent coating. (e) Spray-coated film is flexible and bends easily. Figure 2: α-ZrP nanoplatelets and spray-coated films. ( a ) Transmission electron microscopy (TEM) of α-ZrP nanoplatelets with average size of 100±51 nm, measured from over 200 particles. Scale bar, 100 nm. ( b ) Atomic force microscopy (AFM) height image shows a nanoparticle with grafted brush layer swollen with butyronitrile exhibiting a hemispherical shape (10 nm thick; inset, height profile of nanoparticle). ( c ) Phase image of the same nanoparticle reveals a stiffer phase in the shape of a hexagon at the base (75 nm wide). Scale bar in b , c represents 50 nm. ( d ) Photographs of PI film (top, thickness 25 μm) and PI film spray-coated with smectic α-ZrP/epoxy (bottom, coating thickness 8 μm), demonstrating a uniform, transparent coating. ( e ) Spray-coated film is flexible and bends easily. Full size image Large-scale assembly of smectic nanoplatelets Images obtained from transmission electron microscopy (TEM) show that α-ZrP/epoxy films containing a volume fraction φ =0.044 of α-ZrP consist of a lamellar phase with individual nanoplatelets uniformly aligned parallel to the substrate ( Fig. 3a ). The mean inter-layer distance was found to be 6.4 nm. The mesoscale structure of the thin films was probed using grazing-incidence small-angle X-ray scattering (GISAXS) [30] , [31] . The alignment of 2D crystals can be determined by the location of the interference peaks on the x-z plane of the 2D diffractogram. Lamellar structures that are aligned parallel to the substrate will display Bragg peaks in the vertical axis ( q z axis). Conversely, peaks appearing in the horizontal plane ( q x axis) indicate perpendicular alignment to the substrate [32] . GISAXS studies of the φ =0.044 smectic α-ZrP/epoxy spray-coated PI film show first and second order Bragg peaks characteristic of a lamellar phase exclusively in the q z axis. The results indicate that the nanoplatelets are aligned parallel to the substrate, with a d -spacing of 6.3 nm, in good agreement with TEM results ( Fig. 3b,c ). Wide-angle X-ray scattering (WAXS) detected multiple higher order (up to the fifth order) Bragg peaks from the smectic phase ( Fig. 3d ). The absence of the (002) peak of stacked α-ZrP [19] confirms that the nanoplatelets are fully exfoliated. Nanoplatelet orientation is also confirmed by polarized optical microscopy (POM) of the cured films coated on PI [33] (see Methods and Supplementary Fig. 1 ). A similar phenomenon was observed with POM of the uncured films that were dried at 40 °C for an hour immediately after spray-coating, which suggests that the nanoplatelets rapidly align following removal of the solvent ( Supplementary Fig. 1f,g ). 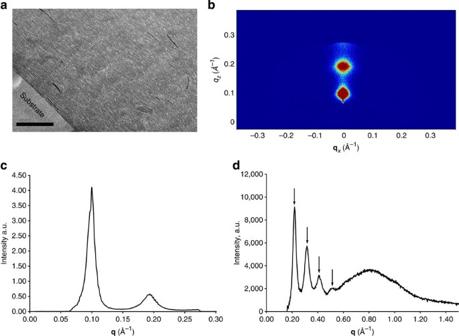Figure 3: Evidence of smectic α-ZrP/epoxy films. (a) TEM of spray-coated film (φ=0.044) shows uniformly aligned nanoplatelets with a mean inter-layer distance of 6.5 nm. Location of substrate is indicated. Scale bar, 200 nm. (b) Grazing-incidence small-angle X-ray scattering (GISAXS) 2D diffractogram with diffractions peaks appearing only along theqzaxis, confirming that nanoplatelets are aligned parallel to the substrate. (c) One-dimensional (1D) diffractogram showing first and second order peaks of smectic phase withd-spacing=6.3 nm. (d) Wide-angle X-ray scattering (WAXS) of film indicates presence of only higher order diffraction peaks (indicated by arrows, second to fifth order) from smectic α-ZrP and a broad amorphous peak. No (002) peaks were detected, which confirms that nanoplatelets are fully exfoliated. The combined data from GISAXS and WAXS confirms the lamellar structure of the nanoplatelet in the coating asq1:q2/q1:q3/q1:q4/q1:q5/q1=1: 2: 3: 4: 5. Figure 3: Evidence of smectic α-ZrP/epoxy films. ( a ) TEM of spray-coated film ( φ =0.044) shows uniformly aligned nanoplatelets with a mean inter-layer distance of 6.5 nm. Location of substrate is indicated. Scale bar, 200 nm. ( b ) Grazing-incidence small-angle X-ray scattering (GISAXS) 2D diffractogram with diffractions peaks appearing only along the q z axis, confirming that nanoplatelets are aligned parallel to the substrate. ( c ) One-dimensional (1D) diffractogram showing first and second order peaks of smectic phase with d -spacing=6.3 nm. ( d ) Wide-angle X-ray scattering (WAXS) of film indicates presence of only higher order diffraction peaks (indicated by arrows, second to fifth order) from smectic α-ZrP and a broad amorphous peak. No (002) peaks were detected, which confirms that nanoplatelets are fully exfoliated. The combined data from GISAXS and WAXS confirms the lamellar structure of the nanoplatelet in the coating as q 1 : q 2 / q 1 : q 3 / q 1 : q 4 / q 1 : q 5 / q 1 =1: 2: 3: 4: 5. Full size image The long-range orientational and positional order characteristic of the smectic organization of nanoplatelets is readily observed even in the bulk nanoplatelet-filled liquid after solvent has been removed. This was verified through large-area TEM imaging ( Supplementary Fig. 2 ) obtained from thin sections of the cured bulk nanoplatelet-filled liquid (see Methods). The evolution of defect structures in the aligned nanoplatelets was captured by electron tomography (ET). Misaligned nanoplatelets were found to be at the origin of disordered zones and showed larger inter-sheet spacing than the surrounding aligned nanoplatelets ( Fig. 4a–e ). A full three-dimensional (3D) ET reconstruction of the nanocomposite confirms that the alignment of the nanoplatelets extends throughout the bulk of the material ( Fig. 4f , Supplementary Movie 1 ). 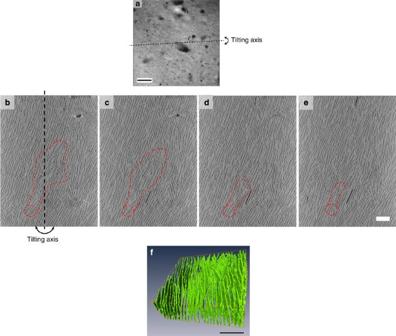Figure 4: ET of α-ZrP/epoxy nanocomposite. (a) Thin section of nanocomposite is rotated along the tilting axis (indicated by dashed line) to capture high-resolution projections that are used to generate tomograms. Scale bar, 200 nm. (b–e) A series of reconstructed tomograms of the nanocomposite; scale bar, 50 nm. Misaligned nanoplatelets form a core (red dashed circles) that disturbs the orderly arrangement of surrounding nanoplatelets. Zones of high disorder originate at the misaligned nanoplatelets with larger inter-sheet spacing (enclosed by red dashed lines). The size of the zone of disorder progressively shrinks as the alignment of core is restored through the thickness of the sample. (f) 3D reconstruction of electron tomography (ET) shows extent of alignment of nanoplatelets (green sheets). Scale bar, 100 nm. The 3D reconstruction confirms that the order persists throughout the bulk of the nanocomposite. A movie (Supplementary Movie 1) of the 3D rendering is available for download online. Figure 4: ET of α-ZrP/epoxy nanocomposite. ( a ) Thin section of nanocomposite is rotated along the tilting axis (indicated by dashed line) to capture high-resolution projections that are used to generate tomograms. Scale bar, 200 nm. ( b – e ) A series of reconstructed tomograms of the nanocomposite; scale bar, 50 nm. Misaligned nanoplatelets form a core (red dashed circles) that disturbs the orderly arrangement of surrounding nanoplatelets. Zones of high disorder originate at the misaligned nanoplatelets with larger inter-sheet spacing (enclosed by red dashed lines). The size of the zone of disorder progressively shrinks as the alignment of core is restored through the thickness of the sample. ( f ) 3D reconstruction of electron tomography (ET) shows extent of alignment of nanoplatelets (green sheets). Scale bar, 100 nm. The 3D reconstruction confirms that the order persists throughout the bulk of the nanocomposite. A movie ( Supplementary Movie 1 ) of the 3D rendering is available for download online. Full size image Gas barrier property of spray-coated films The spray-coated smectic α-ZrP/epoxy films show significant reduction in OTR. Compared with the bare PI films, a 10-fold reduction in oxygen transmission is observed for 7±1 μm thick φ =0.044 α-ZrP/epoxy films. The permeability of individual components in the spray-coated film can be obtained using ideal laminate theory [34] (see Methods). The permeability of the smectic α-ZrP/epoxy coat exhibits more than 20-fold reduction compared with PI and epoxy ( Fig. 5a ). At relative humidity (RH) 0%, the permeabilities of PI, epoxy ( P 0 ) and smectic α-ZrP/epoxy ( P ) films are 7.74, 5.89 and 0.26 cm 3 mm m −2 per day per atm, respectively. At RH 50%, the permeabilities are 4.23, 3.60 and 0.15 cm 3 mm m −2 per day per atm, respectively. At RH 90%, the permeabilities are 3.42, 3.15 and 0.15 cm 3 mm m −2 per day per atm, respectively. Variability in permeability at low- and high humidity levels is low, ~0.1 cm 3 mm m −2 per day per atm. In terms of relative permeability P/P 0 , the values are constant at ~0.04–0.05 at different humidity levels ( Fig. 5b ). Permeability of bare and coated PI films is reduced in the presence of moisture. This reduced permeability is because of water molecules occupying Langmuir sites, which makes them unavailable to oxygen molecules, and the competition between molecular diffusion of water and oxygen [35] , [36] . This stands in contrast to gas barrier films made by the layer-by-layer method, which are particularly sensitive to moisture due to the use of hydrophilic polyelectrolytes. For layer-by-layer films, increases in permeability of 0.2 cm 3 mm m −2 per day per atm and larger have been reported at high humidity levels [37] , [38] . A list of gas barrier films [38] , [39] , [40] , [41] , [42] consisting of clay nanoplatelets/polymer composites prepared using different methods and a comparison of their performance is shown in Table 1 . Although gas barrier films with comparable [42] or substantially lower [38] permeabilities have been reported, it should be noted that none of the previous films possess the unique combination of manufacturability (see Discussion) and performance as the films reported here. Furthermore, the nanoplatelet concentration required to achieve such performance in the current films is significantly smaller than the other films listed in Table 1 . 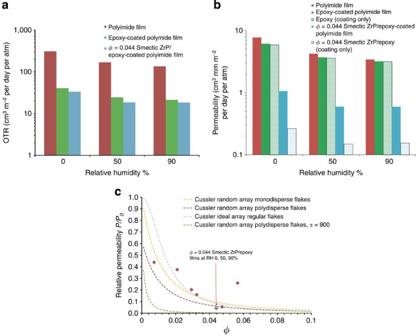Figure 5: Gas barrier property of spray-coated films. (a) Oxygen transmission rate (OTR) of smectic (φ=0.044) α-ZrP/epoxy-coated films tested at three humidity levels (see Methods for details). (b) Permeability of coating was derived from ideal laminate theory. Permeability of smectic α-ZrP/epoxy-coated films shows over 20-fold reduction compared with PI and neat epoxy. (c) Relative permeability of nanocomposite films of various concentrations (diamonds) plotted for comparison with Cussler’s models of permeability of barrier membranes.10,27,28,29Relative permeability of smectic (φ=0.044) α-ZrP/epoxy films is constant at different humidity levels. Except for the green curve, all curves were plotted for nanoplatelets of aspect ratio,α=147. Figure 5: Gas barrier property of spray-coated films. ( a ) Oxygen transmission rate (OTR) of smectic ( φ =0.044) α-ZrP/epoxy-coated films tested at three humidity levels (see Methods for details). ( b ) Permeability of coating was derived from ideal laminate theory. Permeability of smectic α-ZrP/epoxy-coated films shows over 20-fold reduction compared with PI and neat epoxy. ( c ) Relative permeability of nanocomposite films of various concentrations (diamonds) plotted for comparison with Cussler’s models of permeability of barrier membranes. [10] , [27] , [28] , [29] Relative permeability of smectic ( φ =0.044) α-ZrP/epoxy films is constant at different humidity levels. Except for the green curve, all curves were plotted for nanoplatelets of aspect ratio, α =147. Full size image Table 1 Comparison of nanocomposite gas barrier films prepared by various methods. Full size table Many models of the gas barrier effect for polymers filled with flake-like inorganic particles have been proposed based on the assumption that the flakes are oriented perpendicular to the direction of gas flow [10] , [27] , [28] , [29] , [43] . The relative permeability is typically expressed as a function of φ and α (a list of these models are given in Supplementary Table 1 ). Models that include flakes with non-perpendicular orientation allow higher permeation of gas molecules and are not considered here [40] , [41] . The simplest model proposed by Cussler [10] assumes that for a 2D, periodic array of ribbons, the relative permeability is of the form P/P 0 =(1+( μ ¼ × α 2 × φ 2 )/(1− φ )) −1 , where μ is a geometric factor. For an ideal array of regular sized flakes, μ =1. The modified Cussler-Aris model utilizes a more general form of the geometric factor, μ =π 2 / 16 ln 2 (α/2) , derived by Fredickson and Bicerano [27] , to account for strong overlapping of the fillers in the semi-dilute regime. Nielsen’s model is suitable in the dilute regime where there is little or no overlapping of fillers. The Fredickson–Bicerano model is a more sophisticated approximation that collapses to the Nielsen or Cussler–Aris model at certain limits. The Gusev–Lusti model is computationally derived from a finite element model and is considered to more closely describe the real performance of a polydisperse array of isolated plates in an isotropic matrix. Several spray-coated α-ZrP/epoxy films were prepared ( φ =0.007–0.047) and show that permeability decreases with concentration of ZrP ( Fig. 5c ). In Fig. 5c , the concentration-dependent relative permeability is compared with Cussler’s models. A comparison of performance with all of the models mentioned above is provided in Supplementary Fig. 3a . At φ =0.007–0.032, the measured data fall within the expected range of the 2D models proposed by Cussler. At φ =0.044 and 0.047, the Random Array Polydisperse Flakes model [43] gives particularly close predictions to experimental data. At φ =0.057, there is an anomalous increase in permeability, which is discussed in the following paragraph. The substantial improvement in performance of barrier films in this study compared with previous work on α-ZrP/epoxy nanocomposite films by Sun et al. [39] ( Supplementary Fig. 3a ), is attributed to the high degree of order achieved here. Thin-film SAXS studies were carried out using nanocomposite thin films spray-coated on glass plates ( Fig. 6a ). At the lowest filler concentration ( φ =0.007), the thin film is isotropic and shows no diffraction peaks. Diffraction peaks indicative of lamellar structure appear with increasing strength as concentration increases from φ =0.021 to 0.032. At φ =0.044 and higher, the diffraction peaks dominate the background signal that shows that the lamellar structure is of sufficient order to cause high-intensity Bragg reflections. The inter-layer d -spacing shows a corresponding decrease with increasing nanoplatelet concentration in the spray-coated films ( Fig. 6b ). With the exception of φ =0.057, the decrease in inter-layer separation is well correlated with the decrease in gas permeability, which verifies the physical basis for the tunable gas barrier effect. The anomalous behaviour at φ =0.057 is possibly a result of matrix degradation from the longer heating time and higher temperature required to fully cure the highly filled epoxy. A second explanation is that the self-ordering ability of the nanoplatelets is reduced at very high volume fractions owing to the higher viscosities of the nanoplatelet-filled epoxy ( vide infra ). TEM of thin films at the concentration φ =0.047 and 0.057 shows that while the smectic arrangement is maintained, topological defects are observed at higher volume fraction ( Fig. 6c,d ). The observation of s =½ disclinations in Fig. 6d suggests that there is a coexistence of nematic and smectic phases. The presence of such defects provides an easier path for gas diffusion in the film and thereby effectively diminishes gas barrier property. The inter-layer distances (6.4, 6.6 and 6.8 nm for φ =0.044, 0.047 and 0.057 films, respectively) measured from electron micrographs show an increasing trend, as opposed to that observed in SAXS studies that show decreasing d -spacing at higher volume fractions ( Fig. 6b ). This is attributed to an increase in the number of defects in the layers. The presence of defects is not captured directly in the SAXS data, as only regularly spaced smectic layers produce sharp diffraction peaks. Consequently, while the smectic layers show smaller d -spacings, inter-layer distance in the overall film will be increased because of the greater disorder of nanoplatelets. 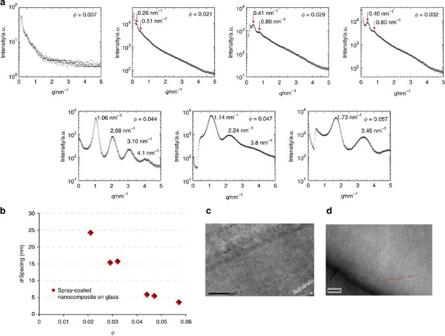Figure 6: Evolution of smectic structure in spray-coated films. (a) Evolution of one-dimensional (1D) SAXS pattern of thin films on glass with increasing nanoplatelet concentration. Peaks positions are indicated when present.φ=0.007 isotropic →φ=0.021–0.032 weak lamellar peaks →φ=0.044–0.057 strong lamellar peaks. (b) Inter-layerd-spacing decreases with increasing nanoplatelet concentration and mirrors the trend seen in the tunable gas permeability of thin films. (c,d) TEM ofφ=0.047 and 0.057 films, respectively. Scale bars, 200 and 100 nm, respectively. Mean inter-layer distances were found to be 6.6 and 6.8 nm, respectively. A disclination of strengths=1/2 (indicated by red arrow) is observed in theφ=0.057 film. Figure 6: Evolution of smectic structure in spray-coated films. ( a ) Evolution of one-dimensional (1D) SAXS pattern of thin films on glass with increasing nanoplatelet concentration. Peaks positions are indicated when present. φ =0.007 isotropic → φ =0.021–0.032 weak lamellar peaks → φ =0.044–0.057 strong lamellar peaks. ( b ) Inter-layer d -spacing decreases with increasing nanoplatelet concentration and mirrors the trend seen in the tunable gas permeability of thin films. ( c , d ) TEM of φ =0.047 and 0.057 films, respectively. Scale bars, 200 and 100 nm, respectively. Mean inter-layer distances were found to be 6.6 and 6.8 nm, respectively. A disclination of strength s =1/2 (indicated by red arrow) is observed in the φ =0.057 film. Full size image The relative permeability as a function of aspect ratio was plotted for φ =0.044 and compared with actual data ( Supplementary Fig. 3b ). Depending on the specific model, the predicted aspect ratio can range from 200 to 2,000. Most of the models fail to give close predictions, which is probably a consequence of individual dispersion of plates being explicitly assumed—an asption that becomes invalid when strong overlapping occurs such as in a highly ordered smectic arrangement of α-ZrP nanoplatelets. An interesting outcome from the Random Array Polydisperse Flakes model is that for α =900 (which can be easily achieved using D =612 nm nanoplatelets), the model predicts a similar gas barrier performance at just φ =0.008, or a 10-fold reduction in permeability at φ =0.03 ( Fig. 5c ). Actual gas barrier performance will likely depend on the ability of nanoplatelets to maintain smectic order at larger aspect ratios. Discotic suspensions are known to go through distinct phase changes that include isotropic (I), nematic (N), columnar (C), smectic (S) and crystalline (X). Typically I-N and N-C transitions are observed for small to moderate aspect ratios α . Theoretical studies have shown that as aspect ratio increases, colloidal discs show I-N transitions at progressively lower volume fractions [44] . Direct I-C transitions can be observed at high volume fractions [45] . Smectic phases are rarely seen and tend to appear only at very high volume fractions [8] or when there is significant polydispersity in the lateral dimension of the colloidal discs [46] . In other situations, smectic phases can be observed when there are long-range repulsive interactions between nanoplatelets that act to stabilize the ordered layers even at very low volume fractions [6] . The appearance of the smectic phase in the epoxy occurs at a significantly lower volume fraction ( φ= 0.021) than an aqueous dispersion of large aspect ratio α-ZrP ( φ= 0.059, α= 2,900) (ref. 46 ) and approaches the volume fraction for the expected I-N transition, which has been observed to be φ~0.02 (for nanoplatelets with α ~150) in aqueous suspensions [44] . Unlike the purely thermodynamically driven self-assembly process in these mildly viscous aqueous solutions, which typically takes several days to complete, the smectic phase observed here in highly viscous epoxy must have formed through a different process as it appears within an hour after the solvent has evaporated. As long-range electrostatic repulsive interactions are not a major factor here (dielectric constant of epoxy is typically 3–4 (ref. 47 ), which is too low for significant accumulation of charges on the nanoplatelet surface), processes that are dependent on such interactions can be ruled out. Surface tension driven self-assembly of colloidal particles at the liquid–air [31] , [48] , [49] and liquid–liquid interfaces [30] have been reported, but these are often slow processes that produce ordered assemblies limited to the interfacial region. Instead, the sterically stabilized nanoplatelets of this work form liquid crystalline phases throughout the solvent-free epoxy liquid [9] , [50] , [51] . This is demonstrated by the bulk liquid epoxy containing φ= 0.040 of sterically stabilized α-ZrP ( Fig. 7a ). Even after the diluent solvent has been completely removed, the liquid shows strong birefringence when observed through crossed-polarizers. When sandwiched between two glass plates, the so-called ‘smectic liquid’ can be induced to display band-like structures ( Fig. 7b ), which are commonly observed in liquid crystalline polymers [52] . In the current context, these structures are believed to be the result of local rotation of nanoplatelets to preserve local order while global order relaxes ( Supplementary Fig. 4a ). SAXS images of the smectic liquid show strong orientation ( Supplementary Fig. 4b ) and peaks characteristic of the lamellar structure, with d -spacing found to be 17.1 nm ( Supplementary Fig. 4c ). The smectic liquid displays extreme shear thinning ( Fig. 7c ), where steady shear viscosity can be reduced by as much as six orders of magnitude at 25 °C and moderate shear rates (~10 2 s −1 ) for φ> 0.040. The extreme shear thinning property of smectic liquid allows for preparation of bulk nanocomposite samples (see Methods; Supplementary Fig. 5a–c ). The SAXS measurements show a slight decrease in d -spacing to 15.2 nm after curing ( Supplementary Fig. 5d,e ), which is consistent with matrix shrinkage during the curing of epoxy. POM images of thin sections prepared from the cured nanocomposite reveal a visually distinctive skin-core morphology, with the skin showing high uniformity in colour and the core showing a complex banded texture ( Fig. 8a ). The general orientation of the normal axis of the nanoplatelets was confirmed to be parallel to the sample stage by insertion of a retardation plate in the optical pathway and observing the change in interference colours [53] ( Fig. 8b–f ). The uniform colours displayed in the skin region are evidence that the nanoplatelets are oriented uniformly parallel to the glass mould that it was in contact with during casting. This observation shows clearly that the substrate has a significant role in aligning the nanoplatelets. 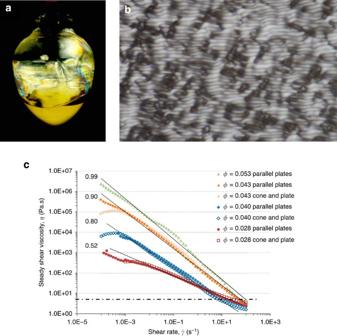Figure 7: Smectic (φ=0.040) α-ZrP/epoxy liquid. (a) The liquid shows strong birefringence, when photographed between cross-polarizers. (b) Polarized optical microscopy (POM) of liquid sandwiched between two glass plates shows banded structures. Scale bar, 10 μm. (c) Extreme shear thinning with increasing shear rate is observed from the measurements of steady shear viscosity for the α-ZrP/epoxy liquids. Viscosity of the liquids show as large as six orders of magnitude reduction. Numbers on the left of curves indicate the exponent value,n(given by ), which approaches unity as α-ZrP concentration increases. Dash-and-dot line indicates the viscosity of neat epoxy~4 Pa·s for comparison. Figure 7: Smectic ( φ =0.040) α-ZrP/epoxy liquid. ( a ) The liquid shows strong birefringence, when photographed between cross-polarizers. ( b ) Polarized optical microscopy (POM) of liquid sandwiched between two glass plates shows banded structures. Scale bar, 10 μm. ( c ) Extreme shear thinning with increasing shear rate is observed from the measurements of steady shear viscosity for the α-ZrP/epoxy liquids. Viscosity of the liquids show as large as six orders of magnitude reduction. Numbers on the left of curves indicate the exponent value, n (given by ), which approaches unity as α-ZrP concentration increases. Dash-and-dot line indicates the viscosity of neat epoxy~4 Pa·s for comparison. 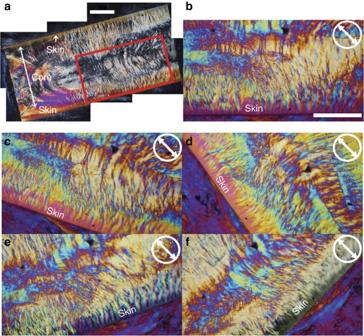Figure 8: Smectic (φ=0.044) α-ZrP/epoxy bulk nanocomposite. (a) Composite image of the individual polarized optical micrographs for smectic α-ZrP/epoxy nanocomposite observed in the direction parallel to the glass mould and perpendicular to the flow direction of the epoxy. Scale bar, 1 mm in botha,b. The difference in texture in the skin and core is apparent, with the skin showing high uniformity in colour and the core showing a complex banded texture. (b–f) Observation via POM with a retardation plate of Γ=530 nm inserted in the optical pathway, oriented in the north-east direction (indicated by the circle and double arrow located upper right corner). The region under observation is demarcated by the red box ina. The sample was oriented at the angles (b) 0°, (c) −20°, (d) −45°, (e) 20° and (f) 45°. Ind, the observed region shows a bright yellow colour, especially in the skin region, which indicates relatively high birefringence and subtractive retardation. Inf, the same region shows a dark yellow-green colour, indicating low birefringence and additive retardation. The results demonstrate that the nanoplatelets are aligned perpendicular to the sample stage on average53. The POM results are consistent with nanoplatelets in the skin region being aligned parallel to the glass mould. Full size image Figure 8: Smectic ( φ =0.044) α-ZrP/epoxy bulk nanocomposite. ( a ) Composite image of the individual polarized optical micrographs for smectic α-ZrP/epoxy nanocomposite observed in the direction parallel to the glass mould and perpendicular to the flow direction of the epoxy. Scale bar, 1 mm in both a , b . The difference in texture in the skin and core is apparent, with the skin showing high uniformity in colour and the core showing a complex banded texture. ( b – f ) Observation via POM with a retardation plate of Γ=530 nm inserted in the optical pathway, oriented in the north-east direction (indicated by the circle and double arrow located upper right corner). The region under observation is demarcated by the red box in a . The sample was oriented at the angles ( b ) 0°, ( c ) −20°, ( d ) −45°, ( e ) 20° and ( f ) 45°. In d , the observed region shows a bright yellow colour, especially in the skin region, which indicates relatively high birefringence and subtractive retardation. In f , the same region shows a dark yellow-green colour, indicating low birefringence and additive retardation. The results demonstrate that the nanoplatelets are aligned perpendicular to the sample stage on average [53] . The POM results are consistent with nanoplatelets in the skin region being aligned parallel to the glass mould. Full size image The large discrepancy in d -spacings of bulk liquid (17.1 nm) and spray-coated films (6.3 nm) appears puzzling at first. This, however, can be resolved upon careful analysis of the formation process of the smectic phase. The nanoplatelet-filled spray solution does not exhibit any liquid crystalline phases, which was verified by the absence of birefringence in the quiescent solution placed between crossed polarizing films. Upon spraying, the smectic phase is most likely initiated at the substrate/solution interface and the solution/air interface, where the nanoplatelets can most easily align parallel to the interface. As solvent is removed, the increasing concentration of nanoplatelets rapidly forces them to self-organise from random configuration ( Fig. 9a ) into nematic and smectic regions ( Fig. 9b ), and may possibly be aided by shear generated during solvent evaporation. Depletion interactions have been known to induce formation of liquid crystalline phases at low volume fractions in colloid/polymer mixtures, which could be a significant factor here, if the epoxy pre-polymer is large enough to enhance the excluded volume effect [54] , [55] . In spray-coated films, it is proposed that the lowest d -spacing achievable is limited by the height of the brush layer in epoxy (brush height depends on solvent environment and thus is not equivalent to the brush height reported in Fig. 2b ), leading to a layer of highly concentrated nanoplatelets ( φ=t/d= 0.68/6.3=0.108). In the bulk liquid, this alignment and organization process will continue as further vaporization of solvent and continuous rotation of the flask provides shearing forces throughout the liquid ( Fig. 9b ). This also has the effect of expanding the d -spacing as shear flow induces epoxy to enter the space between nanoplatelet layers. The relatively high viscosity of epoxy suppresses the randomizing effects from Brownian motion of the shear-aligned nanoplatelets, further contributing to the stability of the smectic layers [56] , [57] , [58] . Consequently, the d -spacing relation for lamellar structure φ=t/d, which predicts that φ= 0.040 for d =17.1 nm and t =0.68 nm ( Fig. 9c ), is in excellent agreement with measured φ for the bulk liquid. This suggests that a homogeneous dispersion has been achieved. In the bulk liquid, the shear thinning behaviour and elevated temperature where this takes place are believed to favour the seemingly contradictory tendencies to align the nanoplatelets and homogenize their distribution. 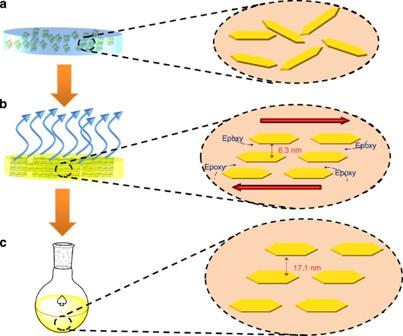Figure 9: Formation process of smectic phase in (φ=0.040) α-ZrP/epoxy liquid. (a) The nanoplatelets initially assume random orientation in the dilute acetone solution. (b) Nanoplatelets are aligned by shear (red arrows) generated as solvent vaporizes on the liquid surface. This aligned surface layer is highly concentrated and the nanoplatelets assemble into smectic phase with smalld-spacing (d=6.3 nm). (c) Further vaporization of solvent and continuous rotation of the flask provides constant shearing throughout the liquid. This has dual effect of inducing alignment of nanoplatelets and expandingd-spacing as epoxy flows between nanoplatelet layers. All solvent is completely removed through the process and thorough homogenization of the liquid results in smectic phase withd=17.1 nm, in agreement with the expected values at this concentration of nanoplatelets (φ=t/d=0.68/17.1=0.04). Figure 9: Formation process of smectic phase in ( φ =0.040) α-ZrP/epoxy liquid. ( a ) The nanoplatelets initially assume random orientation in the dilute acetone solution. ( b ) Nanoplatelets are aligned by shear (red arrows) generated as solvent vaporizes on the liquid surface. This aligned surface layer is highly concentrated and the nanoplatelets assemble into smectic phase with small d -spacing ( d =6.3 nm). ( c ) Further vaporization of solvent and continuous rotation of the flask provides constant shearing throughout the liquid. This has dual effect of inducing alignment of nanoplatelets and expanding d -spacing as epoxy flows between nanoplatelet layers. All solvent is completely removed through the process and thorough homogenization of the liquid results in smectic phase with d =17.1 nm, in agreement with the expected values at this concentration of nanoplatelets ( φ=t/d= 0.68/17.1=0.04). Full size image The stability of the smectic mesophases of α-ZrP in epoxy, at lower than expected volume fractions, suggest that there may possibly be broader application of this technology in the manufacture of liquid crystalline materials. The rheology of the smectic epoxy liquid is favourable to large-scale manufacturing of both bulk and fibre materials. Feature sizes <10 nm are easily reproduced without the need of any sophisticated machinery or a clean room environment, in sharp contrast to photolithography. The short period of time required for nanoplatelets to self-assemble over any surface is critical to practical applications, providing an enormous advantage over other methods of making nanocomposite-based gas barrier films. Highly oriented films can be spray-coated under normal environment without taking any special precautions; making this a highly flexible manufacturing technique. The broad applicability of the grafting mechanism used here allows a wide selection of functional 2D crystal materials to be available for incorporation into polymer matrices. This technology promises to be of interest to fields as diverse as electronics, catalysts, environmental and composite materials. Clay-based gas barrier films have been shown to be outstanding flame retardant materials, and the reported technology is expected to produce similar performance [59] . The manufacture of highly selective separation membranes in particular can benefit from this technique, where in principle, smectic zeolite nanosheets could efficiently select the molecules that permeate through the membranes [60] . It should be noted that the reported technology is not restricted to cured films, as it was shown that orientation occurs rapidly after solvent is removed. The appropriate selection of the liquid phase can lead to a stable material with useful optical properties like iridescence [6] , [61] , [62] , and which may be activated by an electrical or magnetic field through an electrically or magnetically active 2D crystal material. Materials Zirconyl chloride (ZrOCl 2 8H 2 O, 98%, Sigma-Aldrich), phosphoric acid (85%, EM Science) and acetone (ACS grade, EMD) were used as received. A commercial polyoxyalkyleneamine, (chemical structure, H 3 C(OCH 2 CH 2 ) 19 (OCH 2 CHCH 3 ) 3 NH 2 ) Jeffamine M1000 with a reported average molecular weight of 1,000 was received as a gift from Huntsman Chemical. Bisphenol F epoxy (EPON 862) and Epikure W curing agent were purchased from Momentive. Preparation and exfoliation α-ZrP This procedure produces α-ZrP nanoplatelets with a nominal size of 100 nm. A sample of 20.0 g ZrOCl 2 8H 2 O was refluxed with 200.0 ml 3.0 M H 3 PO 4 in a Pyrex glass flask at 100 °C for 24 h. After the reaction, the products were washed and collected by centrifugation three times. Then, the α-ZrP was dried at 65 °C for 24 h. The dried α-ZrP was ground with a mortar and pestle into fine powder. Exfoliation was carried out using M1000. A sample containing 0.5 g α-ZrP was weighed and dispersed in 25 ml acetone by sonication for 30 min. A 0.6 g ml −1 solution of M1000 in acetone was prepared. A volume of 2.77 ml M1000 solution was added dropwise to the stirring α-ZrP dispersion. The dispersion was stirred for 4 h then sonicated for 60 min, followed by centrifugation at 10,000 r.p.m. for 30 min in polytetrafluoroethylene tubes (Nalgene Oakridge, Thermo Scientific). The sediment was removed leaving a clear suspension containing only exfoliated α-ZrP and excess polyoxyalkyleneamine. The clear suspension was centrifuged at 20,000 r.p.m. for 2 h (Sorvall Evolution RC, Thermo Scientific) and the exfoliated α-ZrP was collected as a gel while the excess polyoxyalkyleneamine remained in the supernatant. The exfoliated α-ZrP was redispersed in 25 ml acetone. Preparation of α-ZrP/epoxy bulk nanocomposite Bisphenol F epoxy was dissolved in 12 ml acetone and added dropwise to the stirring exfoliated α-ZrP dispersion. The dispersion was allowed to stir for 4 h and the solvent was removed in a rotary evaporator at an elevated temperature to form a clear, viscous liquid with a dark yellow tint. Curing agent W (26.4 phr) was added to the α-ZrP/epoxy liquid, which was then heated to 80 °C and mixed in a rotary evaporator. The marked shear thinning property of the smectic liquid allows films to be cast in an upright glass mould.The liquid was poured into a vertical glass mould and cured at 80 °C for 100 min, 120 °C for 120 min and 177 °C for 120 min to form a bulk nanocomposite plate. A section of the nanocomposite, taken in the direction parallel to the flow direction of the epoxy, was cut and polished. The process is illustrated in Supplementary Fig. 5a–c . Preparation of α-ZrP/epoxy solution This procedure yields a nanocomposite with 10 wt% ( φ =0.044) α-ZrP. Bisphenol F epoxy (2.33 g; EPON 862, Momentive) was dissolved in 5 ml acetone to form a clear solution. The epoxy solution was added dropwise to the stirring dispersion containing 0.5 g α-ZrP. The dispersion was allowed to stir for 4 h. The solution was concentrated to obtain a 20 wt% solution. Curing agent W (0.62 g; Epikure W, Momentive) was added to the solution and homogenized by stirring. Spray-coating of α-ZrP/epoxy onto substrate film The α-ZrP/epoxy solution was loaded into an airbrush style spray-gun (Master Airbrush G444-SET, needle nozzle 0.5 mm and Royal Mini Air Compressors, TC-20B, flow rate 23 l per min) and sprayed onto a substrate of PI film (Apical, Kaneka) with a thickness of 25 μm or glass microslides (VWR, thickness 1 mm). The solution was manually sprayed multiple times onto the substrate to achieve the desired film thickness. The solutions with lower concentration α-ZrP require a thicker coat to form a continuous layer because of the poor spreading ability of epoxy at raised temperatures. The spray-coated PI film was dried in an oven at 40 °C for 1 h. For the concentrations φ =0.007, 0.021, 0.029, 0.032 and 0.044, the nanocomposite was cured at 120 °C for 2 h, 177 °C for 4 h and 200 °C for 4 h. An additional step of 240 °C 4 h or 240 °C 6 h was required for φ =0.047 and 0.057, respectively, to achieve full cure. The thickness of the cured nanocomposite coatings ranged from 7 to 44 μm. In particular, the thickness of coatings with concentrations φ =0.044–0.057 range from 7 to 13 μm. The thickness of the spray-coated films was measured using a dial gauge (Mitutoyo) and the average of six readings was recorded. Neat epoxy does not form a continuous coat via spray-coating; instead, the bar-coating technique was used. Bisphenol F epoxy (15 g) was mixed with 3.92 g curing agent W homogenized in a rotor-evaporator under reduced pressure and heat. The mixture was heated to 120 °C for 30 min until a viscous consistency is reached. The viscous mixture was applied onto heated (60 °C) PI films laid onto mould-release paper using a film coater (Elcometer 4340). The film was cured at 120 °C for 2 h and 177 °C for 2 h. The average thickness of the coats was measured to be 127±15 μm. Thermogravimetric analysis The volume fraction of α-ZrP in epoxy was determined by converting mass fraction measured via thermogravimetric analysis using a TA instruments Q500. The samples were heated to 900 °C in air at a heating rate of 20 °C per min and held at 900 °C for 60 min. The solid residue that remains is zirconium pyrophosphate (ZrP 2 O 7 ), which can be converted to the equivalent α-ZrP mass fraction via stoichiometric calculations (mass ratio ZrP/ZrP 2 O 7 =1.136) Mass fraction is converted to volume fraction by using v i =m i /ρ i /∑ m i /ρ i , where m i and ρ i are the mass fraction and density of each component, respectively, in the liquid mixture or nanocomposite. Volume fractions reported are based on inorganic ZrP mass exclusively. Gas permeability of spray-coated films OTR of the films was evaluated using a MOCON OX-TRAN 2/21 in accordance to ASTM D3985. All measurements were carried out at a temperature of 23 °C. A total of four spray-coated films were evaluated for OTR at relative humidities of 0, 50 and 90% for the φ =0.044 α-ZrP/epoxy nanocomposite. At all other concentrations, OTR measurements were performed using two films for each concentration at a RH of 50%. In the ideal laminate theory (ILT), the permeability of the individual lamina is related to the laminate permeability, P ILT =(φ c /P c +φ s /P s ) − 1 , where φ c and φ s are the volume fractions of coating and substrate, respectively. P c and P s are the permeabilities of coating and substrate, respectively. Transmission and POM An Eclipse E400 (Nikon) microscope was used for transmission and POM experiments. Cross-sections of coated films were prepared by mounting cut films onto glass microslides with clear epoxy (Permapoxy 5 min) and polished with abrasive paper to a smooth finish with a thickness of about 50 μm. In thin sections of bulk nanocomposites, the orientation of the normal axis of the nanoplatelets was confirmed to be parallel to the sample stage by insertion of a retardation plate in the optical pathway and observing the change in interference colours [53] ( Fig. 8b–f ). Observation of nanoplatelet orientation Optical microscopy reveals the presence of voids ~3 μm in diameter in the φ =0.044 α-ZrP/epoxy coating ( Supplementary Fig. 1a ), which remarkably does not compromise its gas barrier property. This is explained by the fact that the voids do not form continuous pores through the thickness of the coating. The occurrence of voids is found to be substrate dependent, as evidenced by the void-free coating formed on glass substrate ( Supplementary Fig. 1b ). The formation of voids is a result of the poorer spreading capability of α-ZrP/epoxy over PI. POM of the films coated on PI reveals a featureless black image except at the fringes of the voids where birefringence is observed ( Supplementary Fig. 1c ), while films coated on a glass substrate (not shown) display a completely featureless black image because of the complete absence of voids. This suggests that the nanoplatelets are aligned perpendicular to the direction of observation [33] , in agreement with the GISAXS results. In contrast, cross-sections of α-ZrP/epoxy films coated on PI and glass substrate ( Supplementary Fig. 1d,e ) display strong birefringence which is consistent with nanoplatelets being aligned parallel to the substrate. Similarly, evidence of nanoplatelet orientation is observed in uncured films that were dried at 40 °C for 1 h immediately after spray-coating ( Supplementary Fig. 1f,g ). Rheology The rheology of smectic epoxy liquid was measured via an Ares-G2 rheometer (TA Instruments) using a 50.0-mm, 0.02 rad cone and plate fixture made of stainless steel or 40.0 mm aluminium parallel plates. For parallel plate measurements, the gap was maintained between 1.5 and 2 mm. Rheological measurements were carried out at 25 °C. Atomic force microscopy Tapping-mode AFM was carried out by a Bruker Dimension Icon AFM. The image was acquired in air using a MPP-21120-10 probe (Bruker; tip radius, nominal force constant and resonance frequency are 8 nm, 15°, 3 Nm −1 and 75 kHz, respectively). Highly diluted solutions of nanoparticles were dropped onto a Si wafer cleaned previously by Piranha solution (3:1 37% sulphuric acid and 30% hydrogen peroxide mixture; note: Piranha solution is highly corrosive and exothermic when mixed with organic matter, proper safety precautions should be taken during handling). The samples were diluted to 1 p.p.m. in butyronitrile, dropped onto the cleaned Si wafer and dried at room temperature before scanning. This procedure ensures that the brush layer is swollen by the high boiling point butyronitrile (b.p. 117 °C) to enable measurement of brush layers. TEM and ET TEMs were obtained vi a a JEOL JEM–2010. Mean inter-layer distances were calculated from an average of at least 60 measurements from the micrographs. Ultrathin sections were prepared using a Reichert-Jung Ultracut E microtome. ET experiments were carried out with a JEM2200FS (JEOL, Ltd, Japan) equipped with a eucentric specimen stage and in-column electron energy loss spectrometer, which allowed only elastically scattered electrons to produce each projection. The acceleration voltage was 200 kV. In ET, a series of tilted TEM images (projections) are taken ( Fig. 4a ) and is reconstructed into tomograms by the filtered back-projection algorithm [63] . The tomograms are then stacked to generate a 3D reconstructed image ( Fig. 4b–f ). A movie of the tomograms is available for download online ( Supplementary Movie 1 ). Wide-angle X-ray scattering WAXS experiments were performed on a Bruker D8-Focus Bragg-Brentano X-ray powder diffractometer at the Texas A&M University X-ray diffraction laboratory (Cu Kα radiation, λ =1.54056 Å). Grazing-incidence and small-angle X-ray scattering GISAXS experiments were performed on a Rigaku S-Max 3,000 unit at the University of Houston. Data was collected at a grazing-incidence angle of 0.05 degrees (Cu Kα radiation, λ =1.54056 Å). Small-angle X-ray scattering (SAXS) experiments were performed at the Japan Synchrotron Radiation Research Institute SPring-8 facility located in Hyogo, Japan. Measurements were taken at the BL40B2 beam line [64] using an incident X-ray with a wavelength of 0.07 nm. Scattered X-rays were detected using an imaging plate and a 2,237 mm sample-to-detector distance calibrated by the peaks of collagen. The scattering vector is defined by q =(4π/λ) sin θ, where λ is the wavelength of the X-rays, and 2θ is the angle between the incident X-ray beam and the scattered X-rays. Spray-coated samples on glass plates were analysed in the thin-film condition with incident angle set at 0.16°. How to cite this article: Wong, M. et al. Large-scale self-assembled zirconium phosphate smectic layers via a simple spray-coating process. Nat. Commun. 5:3589 doi: 10.1038/ncomms4589 (2014).